Extraordinary phylogenetic diversity and metabolic versatility in aquifer sediment Microorganisms in the subsurface represent a substantial but poorly understood component of the Earth’s biosphere. Subsurface environments are complex and difficult to characterize; thus, their microbiota have remained as a ‘dark matter’ of the carbon and other biogeochemical cycles. Here we deeply sequence two sediment-hosted microbial communities from an aquifer adjacent to the Colorado River, CO, USA. No single organism represents more than ~1% of either community. Remarkably, many bacteria and archaea in these communities are novel at the phylum level or belong to phyla lacking a sequenced representative. The dominant organism in deeper sediment, RBG-1, is a member of a new phylum. On the basis of its reconstructed complete genome, RBG-1 is metabolically versatile. Its wide respiration-based repertoire may enable it to respond to the fluctuating redox environment close to the water table. We document extraordinary microbial novelty and the importance of previously unknown lineages in sediment biogeochemical transformations. Terrestrial sediments are massive reservoirs of fresh water and organic matter [1] . They also host a large fraction of the Earth’s living biomass [1] , [2] , [3] . In the marine sedimentary environment, microbial metabolism is responsible for both the production and destruction of methane and other carbon compounds, processes that influence discharge of greenhouse gases into the atmosphere [4] , [5] . In the terrestrial environment, sediments provide the structure for aquifers, and microorganisms within them control the turnover of buried organic carbon [6] , influence the speciation, and thus fate and transport of metals, and alter the chemical form of contaminants, such as uranium [7] or arsenic [8] . Despite the many characteristics that make sediments of great interest and importance, comparatively little is known about their microbiology. Metagenomic approaches have opened up new approaches for defining the microbiology of natural environments, yet the methods have not found extensive application to sediments due to the anticipated high complexity of the microbial community. In the current study, we apply shotgun sequencing to whole-community DNA to directly analyse the membership and reconstruct metabolic characteristics for previously unstudied organisms from a contaminated aquifer adjacent to the Colorado River, CO, USA. This aquifer has been intensively characterized as part of an investigation of the potential for acetate addition to stimulate uranium bioreduction [7] , [9] , yet essentially nothing is known about the background sediment community. The Geobacteraceae have been of primary interest because they bloom in response to acetate addition and are known to impact metal speciation [9] ; however, their representation in background sediment is uncertain. Our results demonstrate the utility of high-throughput short-read sequencing for extensive and simultaneous sampling of hundreds of genomes from sediments with very even species abundance levels in which the dominant organism comprises <1% of the community. Results reveal extraordinary phylogenetic and genomic novelty. In the dominant organism, we uncover evidence for enzymatic novelty and respiratory strategies that are likely advantageous for life close to a fluctuating anoxic–oxic interface. Sediment community phylogenetic novelty Poorly consolidated fluvial sands, gravels and silts containing visible organic matter, such as twigs, roots and grasses, were sampled from 5 and 6 m below the ground surface in a sediment aquifer adjacent to the Colorado River, CO, USA ( Methods ). DNA was extracted and sequenced using Illumina technology, sequences assembled, and genomes reconstructed and analysed ( Methods ). Sequence assembly resulted in depths of coverage ranging from 2 × to 58 × coverage for assembled genome fragments of >5 kb in length. This approach yielded average sequence coverage of 28 × and 37 × for the 5 and 6 m samples, respectively. No individual organism comprised more than 1% of any community, an indication of the very high species evenness of this ecosystem ( Fig. 1 and Supplementary Data 1 ). The Pielou’s index evenness score [10] for the 161 highest abundance taxa in the 5 m sample is J ′=0.91, where a value of 1 indicates a perfectly even sample. Although we reconstructed single fragments encoding at least eight ribosomal proteins from organisms comprising as little as 0.03% of the community, the previously described Geobacter species that proliferate upon acetate amendment of the uranium-contaminated Rifle, CO, aquifer [9] remained below the detection limit. This finding emphasizes the strength of selection imposed by acetate addition. 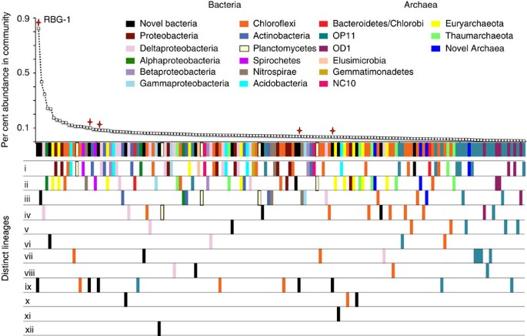Figure 1: Rank abundance and taxonomic affiliations. Top: rank abundance curve for the microbial community in the 5-m depth sample featuring the 161 organisms for which at least 8 of the 16 selected ribosomal proteins (Rpl2, 3, 4, 5, 6, 14, 15, 16, 18, 22, 24 and RpS3, 8, 10, 17, 19) could be recovered. The most abundant organism, RBG-1, represents <1% of the community. RBG-1 lineage members are denoted by red crosses. Bottom: summary of taxonomic affiliations for the 161 community members, based on the concatenated ribosomal protein tree (Supplementary Fig. S1andMethods). The first row denotes the taxonomic assignment of each organism to a phylum or, for the Proteobacteria, class, based on placement and bootstrap support on the tree. Roman numbers i to xii indicate distinct novel clades within each taxonomic division. Novel clades with the same number identifier in different major groups are unrelated. There are 15 new potentially phylum-level groups (i to xii for Bacteria (in black), i to iii for Archaea (in dark blue)). Note that abundance (%) reflects DNA fraction rather than genome copy number (OP11 and OD1 have very small genome sizes). For details, seeMethods,Supplementary Fig. S1andSupplementary Data 1. Figure 1: Rank abundance and taxonomic affiliations. Top: rank abundance curve for the microbial community in the 5-m depth sample featuring the 161 organisms for which at least 8 of the 16 selected ribosomal proteins (Rpl2, 3, 4, 5, 6, 14, 15, 16, 18, 22, 24 and RpS3, 8, 10, 17, 19) could be recovered. The most abundant organism, RBG-1, represents <1% of the community. RBG-1 lineage members are denoted by red crosses. Bottom: summary of taxonomic affiliations for the 161 community members, based on the concatenated ribosomal protein tree ( Supplementary Fig. S1 and Methods ). The first row denotes the taxonomic assignment of each organism to a phylum or, for the Proteobacteria, class, based on placement and bootstrap support on the tree. Roman numbers i to xii indicate distinct novel clades within each taxonomic division. Novel clades with the same number identifier in different major groups are unrelated. There are 15 new potentially phylum-level groups (i to xii for Bacteria (in black), i to iii for Archaea (in dark blue)). Note that abundance (%) reflects DNA fraction rather than genome copy number (OP11 and OD1 have very small genome sizes). For details, see Methods , Supplementary Fig. S1 and Supplementary Data 1 . Full size image To evaluate genomic novelty, we constructed a phylogenetic tree from concatenated alignments of 16 ribosomal proteins (selected based on published metrics of lateral gene transfer frequencies) colocated on single genome fragments [11] , [12] ( Methods ). The resulting tree includes representatives of all genomically sampled bacterial and archaeal phyla ( Supplementary Fig. S1 ). Remarkably, almost every genotype detected was substantially divergent from previously sequenced genomes ( Fig. 1 ). For just the 161 organisms in the 5-m depth sample with sufficient genomic sampling to enable inclusion in Fig. 1 and Supplementary Fig. S1 (a single genome fragment encoding at least 8 of the 16 selected ribosomal proteins), we detect 15 previously genomically unsampled phyla, including 3 clades of archaeal sequences and 12 clades of bacterial sequences (22 distinct sequences total) without clear affiliation to the existing phyla ( Supplementary Data 1 ). We also analysed and classified 317 distinct metagenome-derived 16S rRNA gene sequences ( Supplementary Figs S2–S4 and Methods ). Of these, 50 individual sequences were classifiable only as ‘Bacteria’ or ‘Unclassified Bacteria’. The SILVA classification identified an additional 14 sequences as members of currently genomically unsequenced phyla, including Armantimonadetes (previously Candidate division OP10; 2 sequences), and candidate divisions WS3 (4 sequences), KB1 (1 sequence), OP9 (1 sequence), JL-ETNP-Z39 (1 sequence), GOUTA4 (1 sequence), SM2F11 (1 sequence), TA06 (1 sequence), TM6 (1 sequence) and WCHB1-60 (1 sequence) ( Supplementary Figs S3, S4 and Supplementary Data 2 ). We found that although most of the metagenome-derived 16S rRNA sequences (264 of 317 sequences) share 90–100% identity with publicly available database sequences, the vast majority have <90% identity with genes from genomically characterized organisms (262 sequences). Remarkably, 17 have <76% identity to genes from previously reported genomes ( Supplementary Fig. S2 ). The 16S rRNA gene and ribosomal protein community composition analyses are largely congruent ( Supplementary Fig. S3 ). Notably, in three cases the 16S rRNA and the ribosomal proteins were encoded on the same scaffold, confirming the phylogenetic placement. The 16S rRNA gene-based phylogenetic analysis yielded a tree with lower overall support values compared with the protein tree, as well as occasional erratic placement and long branches for the shorter 16S rRNA genes (not shown). Given the better resolution and consistent topology of the ribosomal protein data set, as well as the use of the protein genes as a more reliable marker for predicted genomic sampling in the metagenome, we rely on the ribosomal protein tree for phylogenetic placements ( Supplementary Fig. S1 ). Overall, all results confirm that we achieved extensive genomic sampling of dozens of new orders, classes and phyla across the bacterial and archaeal domains ( Fig. 1 ). The dominant organism represents a new phylum-level lineage The dominant member of the 5 and 6 m communities is a previously undescribed organism, RBG-1 ( Fig. 1 ). Phylogenetic analysis of RBG-1 and four related genotypes identified from the sediment metagenomes indicates a clade novel at the phylum level. The RBG-1 group forms a highly supported (100/100 bootstrap bipartitions) monophyletic, very deep branching outgroup to the Bacteroidetes/Chlorobi superphylum in the ribosomal protein-concatenated tree ( Fig. 2 ). However, only 12.8% of the predicted proteins in RBG-1 have highest sequence similarity to proteins from this superphylum ( Supplementary Fig. S5A ). Notably, 7.6% of the predicted proteins were most similar to proteins from Caldithrix abyssi ( Supplementary Fig. S5A ), a lineage represented by the single C. abyssi genotype and not currently affiliated with a phylum [13] . The 16S rRNA gene from RBG-1 shares low sequence identity (<83%) to described bacterial phyla, but similar sequences (98% ID) have been detected in a saturated subsurface aquifer in Hanford, WA, USA [14] . The RBG-1 group clusters with low support near the Nitrospirae and Elusimicrobia in the 16S rRNA tree ( Supplementary Fig. 5B ). Given the absence of a stable, supported relationship with a known phylum, ( Fig. 2 and Fig. 3 ), a suggested threshold of 85% 16S rRNA gene sequence identity as a cut-off value for distinguishing new phyla [15] , and the additional support gleaned from numerous protein-coding phylogenetic analyses, we suggest the RBG-1 clade represents a new phylum-level lineage in the domain bacteria. 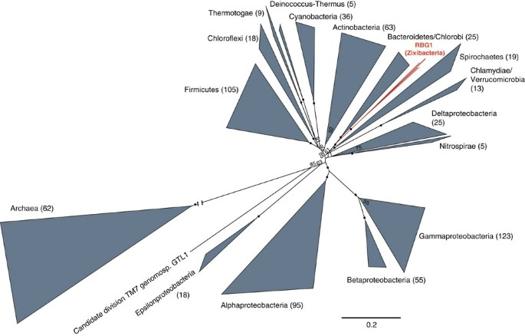Figure 2: Maximum likelihood concatenated 16 ribosomal protein phylogeny. RBG-1 lineage bacteria (now referred to as theZixibacteria phylum) in the 5 m sample are shown in red. Bootstrap support values greater than 55 are displayed, black circles indicate nodes with greater than 95% bootstrap support. Each individual gene data set was aligned using Muscle version 3.8.31 (ref.54) and then manually curated to remove end gaps and single-taxon insertions. The concatenated alignment contained 3,010 unambiguously aligned positions and 1,021 taxa. Maximum likelihood phylogeny was conducted using Phyml56under the LG+α+γ model of evolution and with 100 bootstrap replicates (Methods). Figure 2: Maximum likelihood concatenated 16 ribosomal protein phylogeny. RBG-1 lineage bacteria (now referred to as the Zixibacteria phylum ) in the 5 m sample are shown in red. Bootstrap support values greater than 55 are displayed, black circles indicate nodes with greater than 95% bootstrap support. Each individual gene data set was aligned using Muscle version 3.8.31 (ref. 54 ) and then manually curated to remove end gaps and single-taxon insertions. The concatenated alignment contained 3,010 unambiguously aligned positions and 1,021 taxa. Maximum likelihood phylogeny was conducted using Phyml [56] under the LG+α+γ model of evolution and with 100 bootstrap replicates ( Methods ). 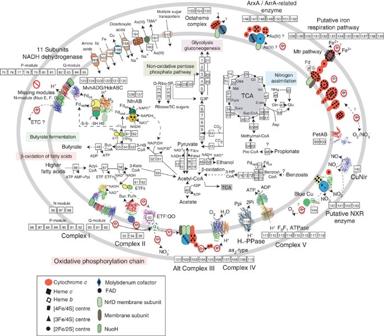Figure 3: Reconstructed energy metabolism of RBG-1. For full gene information and for box numbers seeSupplementary Table S1. Where protein modelling was possible, three-dimensional structural representations are shown (Methods). ArrA, arsenate reductase; ArxA, arsenite oxidase; Blue Cu, blue copper protein; But-CoA, Bbtyryl-CoA; Cit, citrate; CuNir, copper-nitrite reductase;D-ribo-5P,D-ribose-5-phosphate; Fd, ferredoxin; Fum, fumarate; G3P, glyceraldehyde-3-phosphate; 3-HB CoA, 3-hydroxybutyryl-CoA; 3-HP-CoA, 3-hydroxypimelyl-CoA; Iso, isocitrate; 2-oxo, 2-oxoglutarate; 3-Keto CoA, 3-ketoacyl-CoA; Mal, malate; Methylmal-CoA, methylmalonyl-CoA; NXR, nitrite/nitrate oxidoreductase; Oaa, oxaloacetate; Pro-CoA, propionyl-CoA; Suc-CoA, Succinyl-CoA; Succ, succinate. Full size image Figure 3: Reconstructed energy metabolism of RBG-1. For full gene information and for box numbers see Supplementary Table S1 . Where protein modelling was possible, three-dimensional structural representations are shown ( Methods ). ArrA, arsenate reductase; ArxA, arsenite oxidase; Blue Cu, blue copper protein; But-CoA, Bbtyryl-CoA; Cit, citrate; CuNir, copper-nitrite reductase; D -ribo-5P, D -ribose-5-phosphate; Fd, ferredoxin; Fum, fumarate; G3P, glyceraldehyde-3-phosphate; 3-HB CoA, 3-hydroxybutyryl-CoA; 3-HP-CoA, 3-hydroxypimelyl-CoA; Iso, isocitrate; 2-oxo, 2-oxoglutarate; 3-Keto CoA, 3-ketoacyl-CoA; Mal, malate; Methylmal-CoA, methylmalonyl-CoA; NXR, nitrite/nitrate oxidoreductase; Oaa, oxaloacetate; Pro-CoA, propionyl-CoA; Suc-CoA, Succinyl-CoA; Succ, succinate. Full size image Genome and metabolic reconstruction of the dominant organism The reconstructed 2,119,746 bp genome encodes 1,906 protein-coding genes and has 41.9% GC content ( Supplementary Data 3, 4 ). Metabolic predictions indicate that RBG-1 is non-flagellated with a Gram-negative cell envelope. RBG-1 has the genomic potential for respiring a variety of organic compounds (pyruvate, glucose, and possibly acetate and propionate [16] ) as energy and carbon sources, coupled to oxic and anoxic terminal electron acceptors. It has an oxidative tricarboxylic acid (TCA) cycle, near-complete glycolysis/gluconeogenesis pathways and an oxidative phosphorylation pathway ( Fig. 3 and Supplementary Table S1 ). The TCA cycle of RBG-1 includes 2-oxoglutarate ferredoxin oxidoreductase. This enzyme catalyses the reversible oxidative decarboxylation of 2-oxoglutarate to succinyl-CoA and is also a key enzyme of the reductive TCA cycle. However, another key enzyme of this reductive cycle, the ATP-dependent citrate lyase, was not detected in RBG-1 genome, nor were any other key functional genes of other autotrophic pathways [17] ; thus, an autotrophic lifestyle is unlikely in RBG-1. Two key metabolic enzymes of the gluconeogenesis pathway that are highly conserved in archaeal groups have been identified: the bifunctional phosphoglucose/phosphomannose isomerase [18] central to sugar metabolism and a bifunctional fructose 1,6-bisphosphate aldolase/phosphatase proposed to represent an ancestral enzyme [19] ( Supplementary Fig. S6 ). The amino acid sequence of the fructose 1,6-bisphosphate aldolase/phosphatase is highly conserved in archaea and some deeply branching lineages of thermophilic, autotrophic bacteria [19] , but is rare in other bacterial phyla [19] . The presence of glycolytic enzymes with high homology to archaea in RBG-1 may support its phylogenetic position as a deep-branching bacterial lineage, although lateral transfer cannot be ruled out. Typically in bacterial sugar fermentation, ATP is generated by converting acetyl-CoA to acetate using two enzymes (phosphotransacetylase and acetate kinase). However, RBG-1 possesses only a single enzyme (acetyl-CoA synthetase, ADP-forming) for acetate production and ATP generation from acetyl-CoA, a trait shared by fermentative archaea, the early diverging thermophilic bacterium Roseiflexus castenholzii , some obligate syntrophic bacteria [20] and members from the uncultivated bacterial Candidate Division OD1 (ref. 21 ). Homologues of the RBG-1 acetyl-CoA synthetase catalyse the reverse reaction in vitro ; thus, this enzyme might enable RBG-1 to use acetate [22] , [23] . In addition to acetate, RBG-1 can likely produce ATP, butyrate and ethanol from sugar fermentation ( Fig. 3 and Supplementary Table S1 ). When producing butyrate, acetyl-CoA is converted by the action of four enzymes: acetyl-CoA acetyltransferase, NADP-dependent 3-hydroxybutyryl-CoA dehydrogenase (or NAD-dependent hydroxyacyl-CoA dehydrogenase), 3-hydroxybutyryl-CoA dehydratase, NAD-dependent butyryl-CoA dehydrogenase, and the electron transfer flavoprotein complex (ETF) to butyryl-CoA ( Fig. 3 and Supplementary Table S1 ). RBG-1 lacks the typical enzymes involved in converting butyryl-CoA to butyrate present in most fermentative organisms, but analogous to Pyrococcus spp . [22] , may be capable of utilizing the ADP-forming acetyl-CoA synthetase to produce butyrate and generate ATP. In sugar fermentation, the production and consumption of reducing power must be balanced. RBG-1 can regenerate NAD + for glycolysis via butyrate and possibly ethanol production, but lacks lactate- or hydrogen-generating mechanisms. RBG-1 contains several alcohol dehydrogenases and aldehyde dehydrogenases that may have a role in ethanol production ( Supplementary Table S1 ). Genes for the interconversion of pyruvate and ethanol are reversible and directionality is difficult to infer from genomic annotation alone. Thus, in addition to ethanol fermentation, RBG-1 might be capable of respiring ethanol. RBG-1 lacks the RnfA-G complex that facilitates sodium translocation, as well as any H 2 -evolving hydrogenase complexes for reoxidizing reduced ferredoxin produced via pyruvate ferredoxin oxidoreductase and 2-oxoglutarate ferredoxin oxidoreductase enzymes. As a substitute, however, RBG-1 has an alternative 11-subunit NADH dehydrogenase complex I. This complex lacks an NADH-binding module and has been suggested to accept electrons from reduced ferredoxin [24] to produce a proton motive force. Thus, it may be possible that ferredoxin is oxidized via this 11-subunit NADH dehydrogenase. Otherwise, RBG-1 also encodes a NfnAB complex (iron-sulphur flavoprotein complex), which couples the exergonic reduction of NADP + with reduced ferredoxin and the endergonic reduction of NAD + to NADH in reversible reaction [25] ( Fig. 3 ). It has been proposed that under low substrate (ethanol, acetate) concentrations, the NfnAB complex and NADP-dependent 3-hydroxybutyryl-CoA dehydrogenase balance the reducing equivalent budget in Clostridium kluyveri during ethanol-acetate fermentation [25] . The nature of the involvement of alternative complex I and NfnAB complex for reoxidizing ferredoxin is speculative and requires experimental confirmation. Interestingly, we identify a large cluster of genes encoding several ferredoxin-dependent multi-enzyme complexes, including the alternative complex I and the transhydrogenase NfnAB complex mentioned above ( Supplementary Table S1 ). This cluster also includes a cytoplasmic MvhADG/HdrABC hydrogenase complex and its associated maturation system, a pyruvate ferredoxin oxidoreductase and an oxoglutarate ferredoxin oxidoreductase. As RBG-1 lacks coenzyme M and B biosynthetic pathways, the Mvh/Hdr is not likely coupled to reduction of CoM-S-S-CoB with H 2 , as occurs in methanogenesis [26] . The cytoplasmic Mvh/Hdr complex in RBG-1 may function analogously to those in sulphate-reducing bacteria where hydrogen consumption results in oxidative energy generation [27] , [28] . In RBG-1, hydrogen is likely consumed and electrons passed to the 11-subunit NADH dehydrogenase via reduced ferredoxin, resulting in proton motive force generation. Overall, ferredoxin appears important to energy generation in RBG-1. Genes for oxidation of many organic compounds, including short-chain fatty acids (for example, propionate) as well as pyruvate and glucose indicate that RBG-1 is metabolically versatile ( Fig. 3 ). RBG-1 appears capable of metabolizing fatty acids up to a carbon chain length of 16 via β-oxidation to produce acetyl-CoA ( Fig. 3 ) and also has genes involved in the anaerobic degradation of aromatic compounds (for example, benzoate, Fig. 3 , Supplementary Note 1 and Supplementary Table 2 ). Pathway(s) for electron flow during β-oxidation of acyl-CoA intermediates may involve soluble electron transferring flavoproteins (ETFs) and membranous ETF–quinone oxidoreductase (ETF:QO). In mitochondria, ETFs and ETF:QO link oxidation of fatty acids to the mitochondrial oxidative phosphorylation chain [29] . Previous studies showed that syntrophic bacteria, such as Syntrophomonas wolfei , metabolize fatty acids by the β-oxidation pathway. It has been proposed that ETFs may transfer electrons to a membrane-bound FeS oxidoreductase to make H 2 or formate via reverse electron transport [30] . In nitrogen-fixing bacteria, the ETFs and ETF:QO pathway refers to the Fix(ABC) system and has a central role in nitrogen fixation [31] . The Fix system is also implicated in anaerobic carnitine reduction in Escherichia coli [32] . Inspection of the genome of RBG-1 reveals the presence of ETFs and a homologue of the mitochondrial ETF:QO. In the absence of genes required for syntrophy, nitrogen fixation or carnitine reduction, these enzymes might link fatty acid degradation to oxidative phosphorylation encoded by RBG-1. The RBG-1 genome encodes a complete oxidative phosphorylation pathway, with multiple components for some complexes that includes two type-1 NADH dehydrogenase complexes (Complex I), a succinate dehydrogenase (Complex II), a PETAB complex (complex III; cytochrome b -Rieske type complexes, that is, quinol:electron acceptor oxidoreductase), a putative aa 3 -type cytochrome c oxidase (Complex IV) and a F 1 F 0 -type ATPase (Complex V; Fig. 3 and Supplementary Table S1 ). Of interest is an alternative Complex III, ACIII, encoded by at least seven genes ( Supplementary Fig. S7 ). ACIII functionally replaces the bc 1 complex [33] . The ACIII genes cluster with a low oxygen affinity reductase (Complex IV, putative aa 3 -type) and likely form a functional association, as they do in Rhodothermus marinus [34] . RBG-1 lacks high-affinity oxygen reductases ( cbb 3 (ref. 35 ) or bd -quinol oxidases [36] ) suggesting this organism is adapted to higher oxygen concentrations. Overall, the configuration of the oxidative phosphorylation pathway indicates that RBG-1 is capable of aerobic respiration, likely linked to carbon oxidation, including fatty acid oxidation, in the sediment. In the subsurface, bacteria contribute to the global carbon cycle by completely oxidizing organic compounds, such as fatty acids, coupled to sulphate or nitrate reduction [37] . RBG-1 apparently lacks a sulphate reduction pathway, but the genome may encode a nitrite/nitrate oxidoreductase (NXR), a critical enzyme of the nitrification pathway. On the basis of its phylogenetic position within the dimethyl sulphoxide reductase superfamily ( Fig. 4 ), the NXR is related to those identified from Candidatus Kuenenia stuttgartiensis [38] , [39] and Nitrospira defluvii [40] ( Fig. 4 , Supplementary Note 2 and Supplementary Fig. S8 ). In Candidatus K. stuttgartiensis , NXR may facilitate anaerobic nitrite oxidation to nitrate, providing energy and reductant for growth [38] , [39] , whereas NXR in N . defluvii enables growth via aerobic nitrite oxidation [40] . The NXRs of Candidatus K. stuttgartiensis , N. defluvii and the putative NXR from RBG-1 are distinct from those of nitrite oxidizing Proteobacteria ( Nitrobacter or Nitrococcus species [40] ) in that they are oriented towards the periplasm rather than the cytoplasm. The active site facing the periplasm is supported by the presence of a amino-terminal twin-arginine motif via the twin-arginine protein translocation (Tat) pathway. Moreover, it has been suggested that the NXR complex in anammox organisms might also function as a nitrate reductase with small organic compounds as electron donors and nitrate as an electron acceptor [38] , [39] , [41] . A similar role for the NXR complex in RBG-1 cannot be ruled out. If so, RBG-1 could conserve energy via complete anaerobic oxidation of carbon coupled to nitrate reduction, enabling survival under anoxic conditions. Despite the phylogenetic and structural similarity, the catalytic subunit of the putative NXR (α-subunit) of RBG-1 lacks three of the five residues conserved in other nitrate reductases and nitrite oxidoreductases [42] ( Supplementary Fig. S8B ). These residues have been suggested to be involved in substrate binding or to affect the conformation of the substrate entry channel [42] . The RBG-1 enzyme may have a different substrate-binding mechanism and/or substrate, and thus represent a new enzyme type. The genome also encodes a copper-nitrite reductase (NirK), which forms nitric oxide from nitrite. No known nitric oxide reductase is encoded in the RBG-1 genome and, thus, a role for NirK in denitrification seems unlikely; however, a role in anaerobic respiration or detoxification processes cannot be excluded. RBG-1 can assimilate ammonium using glutamate dehydrogenase and glutamine synthetase ( Fig. 3 ). Given the elevated ammonium concentration in the unamended aquifer in the vicinity of the 5 and 6 m sampling locations [43] , these capacities may contribute to the dominance of RBG-1 in the sediment. 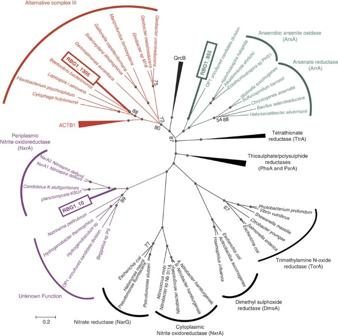Figure 4: Phylogenetic analysis of the catalytic subunits of the dimethyl sulphoxide (DMSO) reductase superfamily. Genes that were newly assigned to the DMSO reductase superfamily (this study) are indicated by boxes. Red circles indicate 100% bootstrap support, green circles indicate nodes with greater than 90% bootstrap support. ACTB1, alternative complex III, domain 1 of subunit B; ArrA, arsenate reductase; ArxA, arsenite oxidase; DmsA, DMSO reductase, alpha subunit; NarG, nitrate reductase, alpha subunit; NrxA, nitrite oxidoreductase, alpha subunit; PsrA/PhsA, polysulphide reductase, subunit A, thiosulphate reductase, subunit A; QrcB, quinone reductase complex, subunit B; TtrA, tetrathionate reductase, subunit A. Accession numbers and amino acid sequences can be found asSupplementary Data 5. Figure 4: Phylogenetic analysis of the catalytic subunits of the dimethyl sulphoxide (DMSO) reductase superfamily. Genes that were newly assigned to the DMSO reductase superfamily (this study) are indicated by boxes. Red circles indicate 100% bootstrap support, green circles indicate nodes with greater than 90% bootstrap support. ACTB1, alternative complex III, domain 1 of subunit B; ArrA, arsenate reductase; ArxA, arsenite oxidase; DmsA, DMSO reductase, alpha subunit; NarG, nitrate reductase, alpha subunit; NrxA, nitrite oxidoreductase, alpha subunit; PsrA/PhsA, polysulphide reductase, subunit A, thiosulphate reductase, subunit A; QrcB, quinone reductase complex, subunit B; TtrA, tetrathionate reductase, subunit A. Accession numbers and amino acid sequences can be found as Supplementary Data 5 . Full size image RBG-1 encodes a previously undescribed oxidoreductase of the dimethyl sulphoxide reductase superfamily ( Fig. 4 ) that is encoded near genes for soluble monoheme/multiheme cytochromes ( Fig. 3 and Supplementary Fig. S7 ). Given its phylogenetic placement with anaerobic complexes, the complex may enable anaerobic growth ( Fig. 4 ). The catalytic α-subunit is divergent from, but forms a two-member clade with, a protein identified from a thermophilic uncultivated member of the Candidate Division OP1 (sharing 42% sequence identity). The RBG-1 and OP1 sequences form a deep-branching addition to the anaerobic arsenite oxidase (ArxA) and arsenate reductase (ArrA) enzyme clades, which is monophyletic with high bootstrap support (93%). ArxA identified in Alkalilimnicola ehrlichii str. is a bidirectional enzyme exhibiting both arsenite oxidase and arsenate reductase activities and is evolutionarily related to arsenate reductase (ArrA) [44] . Amino acid sequence alignment of the α-subunit ( Supplementary Fig. S7 ) revealed a motif for a [4Fe-4S] cluster and a TAT signal peptide similar to that found in ArxA and ArrA. However, the catalytic binding pocket of ArxA and ArrA is not conserved in the RBG-1 catalytic α-subunit ( Supplementary Fig. S7 ), suggesting an alternative binding motif for arsenic compound or another substrate. Taken together, RBG-1 might impact the arsenic geochemical cycle. However, the physiological function of this enzyme complex must be confirmed through experimentation to properly define its function. RBG-1 may have a respiratory pathway for redox transformation of metals, such as iron ( Supplementary Fig. S9 ). The genome encodes the components of a potential Mtr respiratory pathway, which is required for iron reduction in Shewanella species [45] and for iron oxidation by organisms, such as Sideroxydans lithotrophicus and Rhodopseudomonas palustris ( Supplementary Fig. S9 ) [46] , [47] . This raises the possibility that RBG-1 may conserve energy from iron respiration. Candidate genes from RBG-1 for microbial iron respiration are colocated in a gene cluster encoding homologues of Shewanella oneidensis MR-1 MtrA (decaheme cytochrome) and MtrB (outer membrane, porin-type) ( Fig. 3 and Supplementary Fig. S9 ). In iron-reducing Shewanella spp. , MtrAB forms a tight complex localized in the outer membrane where MtrB is proposed to serve as a sheath for embedding MtrA in the membrane [48] . The same structural organization has been proposed for proteins from some iron oxidizers, including S. lithotrophicus and R. palustris [46] , [47] . The gene cluster encoding the Mtr pathway from RBG-1 also encodes two monoheme cytochromes, several multiheme cytochrome c predicted to be periplasmic or localized in the inner membrane, and a PetAB complex (cytochrome b /Rieske complex) ( Supplementary Fig. S9 ). Of note, however, is the lack of homologues of extracellular cytochromes used by Shewanella or Geobacter species for iron oxide reduction, suggesting that mixotrophic ferrous iron oxidation rather than reduction of extracellular ferric iron is the more likely function for this gene cluster (although a function in soluble iron reduction cannot be ruled out). RBG-1 has the machinery and terminal reductases to be capable of iron cycling in oxic and anoxic environments. In addition to the aerobic aa 3 -type cytochrome c oxidase, it is possible that the NXR complex from RBG-1 may function as a nitrate reductase in anaerobic iron oxidation. RBG-1 may grow via nitrate-dependent iron oxidation mixotrophically (with an organic carbon source). In light of these findings, RBG-1 may be capable of iron cycling in both oxic and anoxic subsurface environments. Thus, in addition to multiple carbon degradation pathways, nitrogen-based metabolism, hydrogen consumption, and aerobic heterotrophic growth ( Fig. 3 and Supplementary Table S1 ), we infer that RBG-1 can impact metal biogeochemistry in the sediment. Microbial communities likely contain thousands of different species and can profoundly impact global biogeochemical cycles. However, sediment-associated consortia remain highly understudied. Here we show that cultivation-independent metagenomic approaches can address this knowledge gap. Specifically, we recovered a set of genome fragments, each of which encodes a group of (largely syntenous) ribosomal proteins, and constructed robust phylogenetic trees to classify the more abundant organisms (161 in total). The concatenated ribosomal protein tree approach avoids biases associated with potentially multiple-copy genes (for example, 16S rRNA genes) and, because genes are located on single assembled fragments, the uncertainty introduced by binning. Thus, we could document vast microbial diversity and novelty in the aquifer sediment. Of note, the community largely consists of organisms belonging to bacterial and archaeal phyla, classes and orders not previously recognized or sampled genomically. Not only was it possible to document microbial community structure in a highly complex, even community, our approach yielded a complete genome for the dominant organism, RBG-1. This organism, along with closely related bacteria, defines a new phylum-level lineage, representatives of which can be detected across a range of other environment types. We developed a detailed metabolic model for RBG-1 and discovered evidence for multiple new enzymes and/or biochemical mechanisms. This novelty reflects the substantial evolutionary distance separating RBG-1 from well-characterized organisms. Substantial metabolic versatility could explain the prominence of RBG-1 in aquifer sediments impacted by seasonal fluctuations in the oxic/anoxic boundary resulting from runoff-induced changes in Colorado River discharge. Both the discovery of the RBG-1 lineage and the overall novelty and diversity of its flanking microbial community underline the vast swath of biology that remains to be explored in Earth’s subsurface regions. Field experiment and sample collection The field experiment was carried out in 2007 at the Rifle Integrated Field Research Challenge site adjacent to the Colorado River (Western Colorado, USA). A sediment core was drilled from well D04, in a region not previously impacted by acetate amendments. Sediment samples from 5 and 6 m depths were frozen on site under anaerobic conditions and kept frozen during transport and storage. DNA extraction and sequencing For each depth, 10 independent DNA extractions of 7–14 g of thawed sediment samples were conducted using PowerMax Soil DNA Isolation Kits (MoBio Laboratories Inc., Carlsbad, CA, USA) with the following modification to the manufacturer’s instructions. Sediment was vortexed at maximum speed for an additional 3 min in the SDS reagent, and then incubated for 30 min at 60 °C in place of extended bead beating. The eluted volume was 5 ml per tube, as per the manufacturer’s instructions. DNA was concentrated by sodium acetate/ethanol precipitation with glycogen. Following extraction, precipitation and resuspension, the ten replicate DNA samples were pooled, generating one pooled DNA sample from ~100 g of sediment per depth. Metagenome sequencing was conducted by the Joint Genome Institute. Two rounds of sequencing were done on both samples. Reads from round one were assembled first, and subsequent reassemblies were done using both rounds. For round one (R1), 138,321,556 reads were generated for the 5-m depth sample and 140,430,174 reads for the 6-m depth sample. For round 2 (R2), 359,532,170 reads were generated for the 5-m depth sample and 88,926,182 reads for the 6-m depth sample. The read length for both rounds was 150 bp. Reads were preprocessed using Sickle ( https://github.com/najoshi/sickle ) using default settings to remove low quality bases on both ends of each read. Assembly and annotation Only paired end reads were used in the assemblies. For overall community composition analysis, which focused on the 5-m depth sample, both sequence increments (R1 and R2) for the 5-m depth sample were coassembled using the IDBA_UD assembler under default parameters. The RBG-1 genome was first identified based on its high sequence coverage (~58 × ) in the 5-m (R1) depth sample. The corresponding genotype in the 6-m depth (R1) sample had lower coverage (~21 × ), but assembled into much larger fragments. Scaffolds were binned from the two data sets based on coverage and GC content, and the scaffold sets aligned to each other generated the first draft of the genome. Subsequently, all reads mapping to the draft genome were independently coassembled and the result manually curated. To close gaps in this assembly, we performed an iterative procedure of mapping paired reads to scaffold ends and then reassembling just these reads to bridge scaffolding gaps, as described in Sharon et al. [49] The assembled scaffolds were functionally annotated. Genes were predicted using Prodigal [50] . Amino acid sequences for these genes were then submitted to similarity searches against UniRef90 (ref. 51 ) and the KEGG (Kyoto Encyclopedia of Genes and Genomes) [52] . In addition, UniRef90 and KEGG were searched back against the amino acid sequences to identify reciprocal best-blast matches. Reciprocal best blast matches were filtered at a 300 bit score threshold. One-way blast matches were filtered at a 60 bit score threshold. The amino acid sequences were also submitted to motif analysis using InterproScan [53] . Transfer RNA sequences were predicted using tRNAscan-SE. We ranked the resulting annotations: Reciprocal best-blast matches were ranked the highest, followed by one-way matches, followed by InterproScan matches, followed by hypothetical proteins (just a gene prediction). Concatenated ribosomal protein phylogeny A core group of 16 syntenic ribosomal proteins was selected based on published metrics of lateral gene transfer frequencies (rpL2, 3, 4, 5, 6, 14, 15, 16, 18, 22, 24 and rpS3, 8, 10, 17, 19) [11] , [12] . Reference data sets were derived from the PhyloSift in-house database. The NCBI and Joint Genome Institute IMG databases were mined for the 16 ribosomal proteins from recently sequenced genomes from the Cyanobacteria , Chloroflexi , Nitrospira and TM7 phyla, among others. Scaffolds containing >50% of the 16 genes were identified from the Rifle sediment 5 m depth data set. The identified Rifle ribosomal proteins were searched against the NCBI ‘nr’ database using BLASTp to identify the closest sequenced genome for each sequence, and any genomes not already present in the reference set were added. The complete data set contained 1,021 taxa. Each individual gene data set was aligned using Muscle version 3.8.31 (ref. 54 ) and then manually curated to remove end gaps and single-taxon insertions. Model selection for evolutionary analysis was determined using ProtTest3 (ref. 55 ) for each single gene alignment. The curated alignments were concatenated to form a 16-gene, 1,021 taxa alignment with 3,010 unambiguously aligned positions. A maximum likelihood phylogeny for the concatenated alignment was conducted using PhyML [56] under the LG+α+γ model of evolution and with 100 bootstrap replicates. A total of 161 genotypes were phylogenetically placed: the phylogenetic tree resolves the known phyla and shows that almost every genotype detected was substantially divergent from previously sequenced genomes ( Fig. 1 and Supplementary Fig. S1 ). Taxonomic classification Rifle organisms were classified based on a bootstrap-supported nearest-neighbour methodology of Wu and Eisen [57] . Starting from the immediate ancestor node connecting the Rifle query sequence to a sequenced genome with <70% bootstrap support, and moving toward the root of the tree, the next internal node whose bootstrap support exceeded a 70% bootstrap support cut-off was identified. The common NCBI taxonomy that was shared by all descendants of that node represented the most conservative taxonomic prediction for the query sequence. Exceptions to this were sequences that placed as long branches to the base of phyla were assigned to the affliated phyla given sufficient (>70%) bootstrap support. Sequences most closely associated to phyla with only one sequenced representative (for example, Elusimicrobium , Gemmatimonadetes ) were assigned at the phyla level to those groups. This conservative classification method identified 22 sequences forming 15 distinct clades that were classifiable only to the level of Domain, and which, given the taxon sampling on the tree ( Supplementary Fig. S1 ), are likely representatives of phyla not currently genomically sampled. In addition, 102 sequences forming 37 distinct clades were classifiable to the phylum level but not further, indicating these are additional novel sequences. A minority of sequences could be classified to lower levels of taxonomy: 21, 3, 4 and 9 sequences to the class, subclass, order and family levels, respectively ( Supplementary Data 1 ). Protein phylogenetic analyses Protein tree topologies were inferred using the neighbour-joining method. The distances were computed using the Poisson correction method and are in the units of the number of amino acid substitutions per site. All positions containing alignment gaps and missing data were eliminated based on pairwise sequence comparisons (pairwise deletion option). Phylogenetic analyses were conducted in MEGA5 (ref. 58 ). Protein modelling Three-dimensional structure predictions were generated by the SWISS-MODEL based on protein alignment and secondary structure prediction [59] . SWISS-MODEL is an automated protein homology-modelling server. The alignment mode was utilized for a first approach based on a user-defined target-template alignment. Conservation of key catalytic residues and the secondary structure for each model was confirmed by manual inspection. 16S rRNA gene phylogenetic analyses Phylogenetic placement of RBG-1 was done using a full-length 16S rRNA gene sequence (1,552 bp) derived from the RBG-1 genome. The RBG-1 sequence was included in a 16S rRNA reference gene data set that contained representatives of all known bacterial phyla, candidate phyla sequences identified from the Rifle aquifer [21] , as well as best matches based on alignment of the RBG-1 16S rRNA to Greengenes (environmental and named species) and SILVA (v108) small subunit rRNA databases [60] . The SILVA-derived alignment was masked to remove positions containing only gaps or single taxon insertions and the phylogeny conducted using PhyML under the HKY85+γ model of evolution with 100 bootstrap resamplings. Additional 16S rRNA genes were identified from the RBG community through BLASTn of the metagenome scaffolds against a 16S rRNA reference database. Three hundred and seventeen sequences longer than 600 bp were identified ( Supplementary Fig. S3 ). 16S rRNA genes and fragments were excised from the scaffolds and aligned to the SILVA database using the SINA alignment tool with concurrent classification by the SINA LCA algorithm [60] . All 16S rRNA genes of 600+ bp in length were additionally searched against the NCBI ‘nr’ and ‘refseq_genomic’ databases using BLASTn. Accession codes : Sequences for the rifle sediment metagenome have been deposited at the NCBI Sequence Read Archive (SRA) with Project number BioProject ID# PRJNA167727 , under the accession code SRP013381 . This Whole Genome Shotgun project has been deposited at DDBJ/EMBL/GenBank under the accession AUYT00000000. The version described in this paper is version AUYT01000000. How to cite this article: Castelle, C. J. et al. Extraordinary phylogenetic diversity and metabolic versatility in aquifer sediment. Nat. Commun. 4:2120 doi: 10.1038/ncomms3120 (2013).